Flexible polymer transistors with high pressure sensitivity for application in electronic skin and health monitoring Flexible pressure sensors are essential parts of an electronic skin to allow future biomedical prostheses and robots to naturally interact with humans and the environment. Mobile biomonitoring in long-term medical diagnostics is another attractive application for these sensors. Here we report the fabrication of flexible pressure-sensitive organic thin film transistors with a maximum sensitivity of 8.4 kPa −1 , a fast response time of <10 ms, high stability over >15,000 cycles and a low power consumption of <1 mW. The combination of a microstructured polydimethylsiloxane dielectric and the high-mobility semiconducting polyisoindigobithiophene-siloxane in a monolithic transistor design enabled us to operate the devices in the subthreshold regime, where the capacitance change upon compression of the dielectric is strongly amplified. We demonstrate that our sensors can be used for non-invasive, high fidelity, continuous radial artery pulse wave monitoring, which may lead to the use of flexible pressure sensors in mobile health monitoring and remote diagnostics in cardiovascular medicine. Flexible pressure sensors are essential components in future mobile applications such as rollable touch displays, biomonitoring and electronic skin [1] , [2] , [3] , [4] , [5] , [6] , [7] , [8] , [9] , [10] , [11] . Most of these applications require high sensitivity in the low-pressure regime <10 kPa, fast response time in the millisecond range, and low power consumption. Electronic skin also needs to mimic the sensitivity of human skin over a wide pressure range, with a simple monolithic pressure sensor design enabling cheap large area production. In biomonitoring, pressure sensors are used in continuous pulse and blood pressure recording during surgery or intensive care. Currently, intravascular catheters are used although the infection risk of this invasive method limits its use in newborns and high-risk patients. Therefore, the development of external continuous blood pressure monitoring methods such as arterial tonometry is a field of high research interest [12] . Moreover, analysis of the complete pulse pressure wave form has been shown to provide valuable information for diagnostics of cardiovascular diseases [13] , [14] , [15] , [16] . The high pressure sensitivity requirements have only recently been met by integrated CMOS devices, thus opening the way to a wider spread of arterial tonometry as a routine diagnostic tool [17] , [18] . Flexible and lightweight pressure sensors have the potential to take arterial tonometry even further as they would result in cheap, mobile monitoring devices, making long term diagnostics during normal every-day activities possible. Organic thin film transistors (OTFTs) have been used as transducers for chemical, biological and pressure-sensing devices [19] , [20] , [21] , [22] , [23] , [24] , [25] , [26] . Recently, we reported microstructured polydimethylsiloxane (PDMS) as dielectric layer for flexible capacitive pressure sensors with 0.55 kPa −1 sensitivity and response time in the milliseconds range [3] . In that work, we further demonstrated a new type of active pressure sensor using the microstructured PDMS as gate dielectric for rubrene single crystal field effect transistors. The applied pressure induces a change in the capacitance of the compressible microstructured PDMS dielectric layer, which transduces as the drain-source current changes. The single crystal semiconductor was previously used due to its structural perfection and low surface density of traps yielding devices with very low threshold voltage. However, this device was made on a Si wafer, which makes it not flexible, and also the fabrication and scale-up for practical applications of single crystal devices remain challenging [27] , [28] , [29] . In this communication, we demonstrate a simple process for integration of a microstructured PDMS dielectric in thin film polymer transistors, resulting in highly flexible monolithic transistor devices with unprecedented sensitivity; 15 times higher as compared with the capacitive and single-crystal transistor devices previously reported [3] , >150 times higher than polyvinylidene fluoride piezoresistive sensors [30] , and >20 times higher than commercially available carbon particle-based resistive rubber [2] , [25] , [31] . We achieve this significant increase in sensitivity by operating the transistor in the subthreshold regime where the source-drain current is superlinearly dependent on the pressure-induced capacitance change. Moreover, our sensors show response times in the millisecond range, high stability over >15,000 cycles, and low power consumption <1 mW. As a demonstration of its high pressure and time resolution capabilities, we apply our flexible sensors to continuously monitor the human radial artery pulse wave. Such accuracy was previously only reached with complex instruments such as micromanometers. Device fabrication We fabricated the flexible pressure-sensitive OTFTs by assembling separate layers via lamination ( Fig. 1 ). The first assembly contains bottom source and drain electrodes and the polymer semiconductor on a divinyltetramethyldisiloxane bis(benzocyclobutene) (BCB)-coated polyimide film. Polyisoindigobithiophene-siloxane (PiI2T-Si), a conjugated polymer previously reported by our group [32] , was chosen as the semiconductor because of its high mobility up to 2.45 cm 2 V −1 s −1 and resistance to most solvents as an annealed film. A PDMS layer (thickness 700 nm) coated on top of the PiI2T-Si prevented damage during lamination. Moreover, the good compatibility of the PiI2T-Si with the PDMS protection layer allows for the formation of a homogeneous interface, which is important for the transistor operation and is confirmed by the fact that the transfer curves do not show any significant hysteresis (see below). The second assembly contains the microstructured PDMS dielectric (lines with a triangular cross-section profile with 7 μm height, 7 μm width and 14 μm pitch) on a indium tin oxide (ITO)-coated polyethylene terephthalate (PET) film [3] . Both parts were then laminated in ambient with the two PDMS layers facing each other, and the line structures aligned parallel to the channel. After sealing the edges with epoxy, the device was annealed at 100 °C for 5 h in the glovebox under an inert atmosphere to remove residual water and oxygen. This final annealing step is crucial to ensure good device performance and stability as the polymer semiconductor/PDMS dielectric interface gets doped by oxygen, which leads to poor on–off ratios and large threshold voltage shifts during operation ( Supplementary Fig. S1 ). After annealing, the device was found to be stable over several weeks in ambient (20 °C, 39% r.h.). 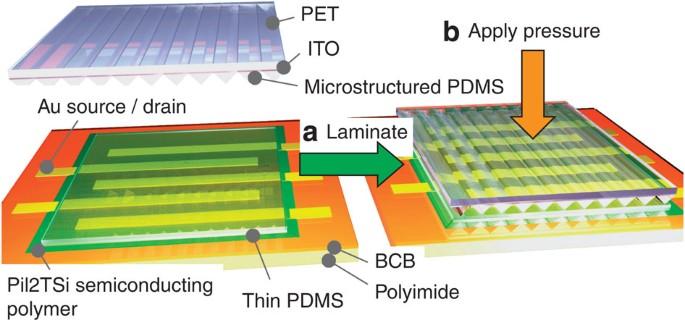Figure 1: Schematic of the final fabrication step of our pressure-sensitive transistor. The sensor is made by laminating two separate layers. The first contains the bottom source-drain electrodes and the semiconducting polymer, and the second contains the gate electrode and the microstructured dielectric. The thin PDMS layer on top of the semiconductor ensures a homogeneous dielectric interface and provides protection during the lamination step. Figure 1: Schematic of the final fabrication step of our pressure-sensitive transistor. The sensor is made by laminating two separate layers. The first contains the bottom source-drain electrodes and the semiconducting polymer, and the second contains the gate electrode and the microstructured dielectric. The thin PDMS layer on top of the semiconductor ensures a homogeneous dielectric interface and provides protection during the lamination step. Full size image Pressure sensor operation Transfer and output characteristics at different pressure loads are given in Fig. 2 . Without a pressure load, the transistor showed a low on–off ratio of 10 due to the low capacitance of the uncompressed PDMS dielectric. Increasing the pressure load to 6.7 kPa resulted in an on-current increase by two orders of magnitude, whereas the off-current slightly decreased. Further increasing the pressure load to 46 kPa increased the on-current by another factor of 2.5 and the on–off ratio increased to 5,000. The output plots showed only partial saturation, which may originate from the presence of unintentional impurity dopants in the channel, probably because most of the device fabrication was carried out in ambient [33] . For all applied pressures, the transfer curves do not show significant hysteresis. 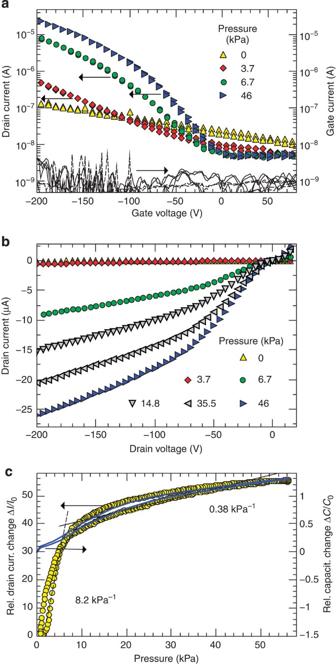Figure 2: Electric characteristics of the pressure sensitive transistor. (a) Transfer curves atVSD=−200 V. (b) Output curves at constantVSG=−200 V. (c) Pressure response of the source-drain current at constantVSD=−200 V andVSG=−200 V and related pressure response of the dielectric capacitance measured at 10 kHz. Forward and backward sweep, that is, pressure increase and decrease, are shown where the higher drain current and capacitance correspond to the backward sweep. Transfer and output curves were taken inside a glovebox with weights placed on the sensor, whereas the high-resolution pressure response measurement incwas performed on an automated z-stage outside the glovebox, resulting in slightly different absolute current changes. Figure 2: Electric characteristics of the pressure sensitive transistor. ( a ) Transfer curves at V SD =−200 V. ( b ) Output curves at constant V SG =−200 V. ( c ) Pressure response of the source-drain current at constant V SD =−200 V and V SG =−200 V and related pressure response of the dielectric capacitance measured at 10 kHz. Forward and backward sweep, that is, pressure increase and decrease, are shown where the higher drain current and capacitance correspond to the backward sweep. Transfer and output curves were taken inside a glovebox with weights placed on the sensor, whereas the high-resolution pressure response measurement in c was performed on an automated z-stage outside the glovebox, resulting in slightly different absolute current changes. Full size image Figure 2 also shows the device current response from 0 to 60 kPa when operated at a constant source drain (−200 V) and source-gate voltage (−200 V). The average pressure sensitivity below 8 kPa was 8.2 kPa −1 . Above 30 kPa, the average sensitivity dropped to 0.38 kPa −1 . When compared with the relative change in the PDMS dielectric capacitance, the saturation current change follows the capacitance change linearly only above about 8 kPa. Below 8 kPa, the relative current change far exceeds the relative capacitance change. While the sensitivity of the capacitive sensor is comparable to what we have reported for line-structured PDMS previously, the strongly enhanced sensitivity in the transistor device deviates from the observations in our previous paper, where we used a rubrene single crystal semiconductor and saw a linear correlation between relative (saturation) current change and capacitance change over the entire pressure regime [3] . The ease of device fabrication with polymer semiconductors and the good device uniformity as discussed later in device array characterizations allowed us to carry out more systematic studies on this effect here. Apparently ( Fig. 2 ), we actually operate the device in the subthreshold regime. In the subthreshold regime, the charge density n s in the channel of a metal oxide semiconductor field effect transistor (MOSFET) is given by with the subthreshold swing parameter and the dielectric capacitance per unit area c a both containing the dielectric capacitance C diel , and V th =kT/q being the thermal voltage, V T the threshold voltage and V the gate voltage [34] . Despite the known differences in operational details between MOSFETs and OTFTs [35] , we can still expect the current in our OTFT device to depend superlinearly on the dielectric capacitance if operated in the subthreshold regime, which matches our experimental observation. The reason for the threshold voltage to be so high at small pressure loads is the combination of a very low capacitance of the structured PDMS dielectric (0.125 nF cm −2 in the uncompressed state) and a non-zero trap density at the polymer semiconductor/PDMS dielectric interface (9.1 × 10 11 cm −2 V −1 , see Methods) where most of the current is flowing [36] , [37] , [38] . This is in contrast to the single crystal device reported previously [3] , which has a much lower threshold voltage because of the use of a rubrene single crystal where interface traps do not have a significant role because the charge conduction channel at low gate voltage reaches deeper into the crystal bulk [35] , [39] . Tuning sensor sensitivity We further investigated how device design and operation parameters influence the sensitivity. Moreover, different applications require sensitivity at different pressure regimes, which makes a general investigation on sensitivity tuning important. We previously reported the effects of the geometry of the PDMS structures and found that pyramid-shaped features were more sensitive to pressure than line-shaped features [3] . Here we report on another geometric aspect, that is, the areal distribution of pyramids, and the influence of transistor source-drain and source gate voltage on the pressure sensitivity. Different from the results presented in Fig. 2 , which were all measured on a device with a line-structured PDMS dielectric (height 7 μm, width 7 μm, spacing 7 μm) we have chosen to investigate four different pyramid structures (height 3 μm, pyramid base width 6 μm, spacing varying from 1.33 to 13.6 μm) in capacitive sensors for the geometrical aspect. The motivation for using pyramids here was to get a more pronounced spacing dependent effect based on the assumption that a higher sensitivity is caused by a higher compressibility per area due to less contact area between the structured dielectric and the top electrode. For the investigations on the influence of source-drain and source-gate voltage on sensitivity, the pyramid structure with 8.85 μm spacing was then incorporated into a transistor device with the same architecture as already described above with the only difference in the channel width being only 4 mm instead of 16 mm. Moreover, as a consequence of the lower height (3 instead of 7 μm), the capacitance of the pyramid structured dielectric was measured to be higher (0.24 nF cm −2 instead of 0.125 nFcm −2 ) which resulted in lower required gate voltages and thus quantitatively different transfer and output characteristics as compared to the device presented in Fig. 2 . 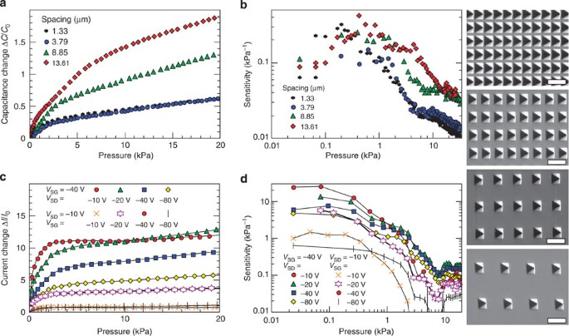Figure 3: Capacitor and transistor pressure sensor sensitivity as a function of design and operational parameters. The first line shows SEM pictures (scale bar, 10 μm) of four different designs of microstructured PDMS: pyramids with 3 μm height and spacing of 1.33, 3.79, 8.85 and 13.61 μm, taken at 45° tilt angle. Graphsaandbshow the relative capacitance change and sensitivity of capacitors with those PDMS microstructures as dielectric. Graphscanddshow the relative current change and sensitivity of a transistor with integrated microstructured PDMS dielectric with 8.85 μm spacing at different transistor source-drain voltages and source-gate voltages. Figure 3 summarizes the results of both studies. For the geometric aspect, we found that a wider spacing resulted in a higher normalized capacitance change and high sensitivity can be maintained at higher pressure regions. While the effect of changing spacing from 1.33 to 3.79 μm is minor, the trend is more obvious going to larger spacings. To further confirm the experimental results, we calculated the capacitance of the investigated structures in an idealized uncompressed state between perfectly parallel electrodes (details see Methods section). It was found that the measured capacitance was always lower, with a larger deviation for a higher spacing (see Supplementary Table S1 ). This deviation could be explained by an additional air gap formed between the PDMS dielectric structures and the top electrode, likely due to the slight curvature of the flexible substrate so that the top and bottom electrodes are not perfectly parallel. We note that the deviation increases with increasing spacing, suggesting that the air gap increases. This is likely due to a smaller contact area between the top electrode and pyramidal structures resulting in less adhesion. As a consequence of the additional air gap, the compression of these structures is actually a superposition of the compression of the air gap against the curved substrate and the compression of the PDMS microstructures. The presence of the air gap may further increase the sensitivity. However, the sensitivity should follow the same trend without the air gap, because in the devices with larger spacings, the applied pressure is distributed over a smaller number of individual pyramids, which therefore get compressed more. In summary, the larger spacing gives rise to two effects, both of which lead to higher sensitivity, that is, an increase in compressibility due to a larger net force onto individual pyramids, and the creation of a larger air gap due to less contact area between the pyramids and the top electrode. Figure 3: Capacitor and transistor pressure sensor sensitivity as a function of design and operational parameters. The first line shows SEM pictures (scale bar, 10 μm) of four different designs of microstructured PDMS: pyramids with 3 μm height and spacing of 1.33, 3.79, 8.85 and 13.61 μm, taken at 45° tilt angle. Graphs a and b show the relative capacitance change and sensitivity of capacitors with those PDMS microstructures as dielectric. Graphs c and d show the relative current change and sensitivity of a transistor with integrated microstructured PDMS dielectric with 8.85 μm spacing at different transistor source-drain voltages and source-gate voltages. Full size image In the transistor configuration, both the source-drain and the source-gate bias voltage were found to have a strong influence on the pressure sensitivity. For the source-drain voltage, a general increase in normalized current change and sensitivity in the low-pressure region (<1 kPa) was achieved by decreasing the bias, for example, the sensitivity at 1 kPa was more than doubled by decreasing the source-drain voltage from −80 to −10 V (1.1 to 2.5 kPa −1 ), whereas at higher pressures, intermediate source-drain voltages around −40 V led to the highest pressure sensitivity. This can be understood as follows. At low pressure, the gate capacitance is low, which causes the transistor to operate entirely in the subthreshold regime, and short-channel effects play an important role, in particular source-drain-voltage-induced injection barrier lowering (transistor transfer curves in Supplementary Fig. S2 ). Therefore, smaller source-drain voltage leads to lower current levels at zero pressure and higher current changes upon pressure increase. At higher pressure, this effect vanishes because the capacitance increases, which reduces short-channel effects, and shifts the transistor operation out of the subthreshold regime. For the source-gate voltage, intermediate values around −40 V consistently resulted in the highest sensitivities over the entire pressure region. This can be understood as follows. Lower source-gate voltage leads to stronger modulation of the subthreshold current by the gate capacitance (see equation (1)). However, at low source-gate voltages, leakage sets a lower limit for the current levels and current changes upon pressure. Therefore, intermediate source-gate voltage leads to the highest sensitivity. Overall, in every pressure region, the normalized current change and thus the sensitivity can be varied by more than one order of magnitude by choosing the appropriate source-drain and source-gate voltage. When comparing the capacitive sensor with the transistor configuration, the largest overall sensitivity amplification is achieved with −40 V source-gate and −20 V source-drain voltage. This driving scheme amplifies the sensitivity of the capacitor by a factor of 50 (0.2–10 kPa −1 ) at low pressure (0.1 kPa) and by a factor of 5 (0.04–0.2 kPa −1 ) at high pressure (10 kPa). Device operation while bent We investigated the device performance while it was bent at different convex curvatures with the tips of the triangular-structured PDMS dielectric facing inward and the line of curvature perpendicular to the channel. We were able to operate the device at all bending radii down to 28 mm, which is far more than required for external biomonitoring applications, for example, attaching the device to a human wrist. We found that the source-drain current was sensitive to the bending radius. 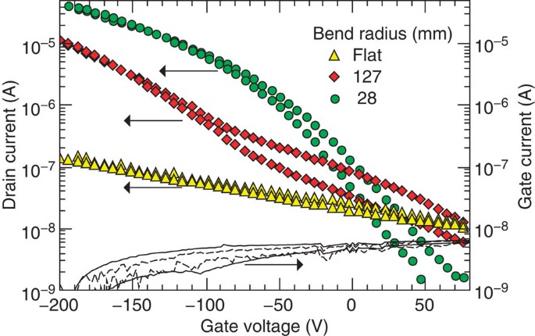Figure 4: Device characteristics while bent. Transfer curves were measured atVSD=−200 V while the device is being attached to objects with different bend radii without applying additional pressure. Figure 4 shows the device characteristics measured at various curvatures. Similar to the low-pressure regime, the transfer curves indicate subthreshold operation at large bending radii with the source-drain current being superlinearly dependent on the inverse of the bending radius. At smaller bending radii, the device operates at above the threshold regime and the source-drain current scales less with decreasing bending radii. Initial device characteristics were recovered after bending ( Supplementary Fig. S3 ). Figure 4: Device characteristics while bent. Transfer curves were measured at V SD =−200 V while the device is being attached to objects with different bend radii without applying additional pressure. Full size image Response time and cycling tests The pressure sensor response time was measured by periodically changing the pressure on the device with a high-precision stepper motor. The source-drain current change was monitored with an oscilloscope via the voltage drop change over a 9-MΩ resistor connected in series with the pressure sensor source at a constant gate and drain voltage of −100 V. Results are given in Fig. 5 . A lower operating voltage at −36 V also resulted in similar characteristics (see Supplementary Fig. S4 ). The operating voltage can potentially be reduced further by using higher dielectric constant elastomers as the dielectric layer. Even with the stepper motor being operated at maximum speed, the pressure sensor showed a virtually instantaneous response to increasing pressure, which was faster than the time resolution of the oscilloscope (<1 ms). The response to pressure decrease was initially delayed by <10 ms, most likely due to the hysteresis effects, which have already been described above. The same set-up was used to investigate the sensor stability to repeated pressure cycling up to >15,000 times, which corresponds to >45 min, during which the transistor was constantly biased at −100 V source-drain and source-gate voltage. 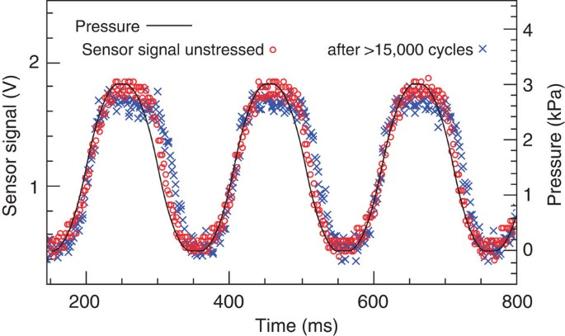Figure 5: Time-resolved sensor response. Periodic fast pressure changes are used to determine the response time taken for the unstressed sensor and after >15,000 pressure cycles (>45 min). Signal is the voltage change measured via a 9-MΩ resistor connected in series to the transistor source. The response time upon pressure increase is instant within the experimental resolution even after cycling stress. The response time upon pressure release is <10 ms for the unstressed sensor and <20 ms after cycling stress. Figure 5 also shows the sensor response after the stress test. It can be seen that the absolute signal has only degraded by <10%. The response upon pressure increase remained constant within the experimental resolution. However, the response time upon pressure release increased from <10 to <20 ms. Figure 5: Time-resolved sensor response. Periodic fast pressure changes are used to determine the response time taken for the unstressed sensor and after >15,000 pressure cycles (>45 min). Signal is the voltage change measured via a 9-MΩ resistor connected in series to the transistor source. The response time upon pressure increase is instant within the experimental resolution even after cycling stress. The response time upon pressure release is <10 ms for the unstressed sensor and <20 ms after cycling stress. Full size image Radial artery pulse measurement As a demonstration of its high fidelity and functionality in a bent state we attached our flexible pressure sensor to an adult human wrist, just above the radial artery as it is usually done in arterial tonometry. The recording set-up was the same as for the response time and cycling tests using an oscilloscope. 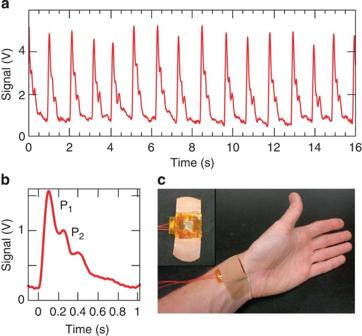Figure 6: Pulse wave of the radial artery measured with our sensor. Data were obtained while attaching the pressure sensor to the wrist of a test person (c). (a) Real-time transient signal. (b) Averaged signal from 16 periods (separate measurements). Source-drain and source-gate voltage was −100 V. The source-drain current was below 10 μA, resulting in a power consumption below 1 mW. The signal was recorded with an oscilloscope as the voltage drop over a 9-MΩ resistor connected in series to the OTFT source. The absolute signal was found to vary strongly with sensor placement location and wrist posture as typically seen in radial tonometry. This also explains the difference in absolute signal strength between the real-time transient signal (a) and an averaged signal (b), which were recorded in two separate measurements. However, the relevant parameters for arterial stiffness diagnostics, that is, the time delay betweenP1andP2, and the radial augmentation index AIr=P2/P1can be determined independent from absolute signal strength. Figure 6 shows a real-time record over several pulse periods, as well as a high-resolution picture of one pulse wave averaged over 16 periods. A characteristic pulse pressure shape was obtained with three clearly distinguishable peaks known to be caused by superposition of the incoming blood wave ejected by the left ventricular and the reflected wave from the lower body [13] . From the first two peaks, P 1 ( t 1 ) and P 2 ( t 2 ), one can easily derive two of the most commonly used parameters for arterial stiffness diagnosis, that is, the time delay between the first and second peaks Δ T DVP = t 2 − t 1 , and the radial augmentation index AI r = P 2 / P 1 (ref. 13 ). For the test person, Δ T DVP =155 ms and AI r =59% have been determined, which are characteristic values expected for a healthy adult male in his mid thirties of age. Moreover, our sensor was able to resolve small features in the diastolic tail of the pulse pressure wave that the majority of sensors used in arterial tonometry do not detect, and hence could potentially be of use for more detailed diagnostics. Figure 6: Pulse wave of the radial artery measured with our sensor. Data were obtained while attaching the pressure sensor to the wrist of a test person ( c ). ( a ) Real-time transient signal. ( b ) Averaged signal from 16 periods (separate measurements). Source-drain and source-gate voltage was −100 V. The source-drain current was below 10 μA, resulting in a power consumption below 1 mW. The signal was recorded with an oscilloscope as the voltage drop over a 9-MΩ resistor connected in series to the OTFT source. The absolute signal was found to vary strongly with sensor placement location and wrist posture as typically seen in radial tonometry. This also explains the difference in absolute signal strength between the real-time transient signal ( a ) and an averaged signal ( b ), which were recorded in two separate measurements. However, the relevant parameters for arterial stiffness diagnostics, that is, the time delay between P 1 and P 2 , and the radial augmentation index AI r = P 2 / P 1 can be determined independent from absolute signal strength. Full size image Array demonstration For electronic skin applications, it is desirable to scale up the sensor to an array configuration of several pixels to collect spatially resolved pressure information. As a demonstration ( Fig. 7 ), we fabricated a 4 × 4 pixel array with a total area of 1 × 1 cm 2 and each pixel having an area of ~1.7 mm 2 including the source-drain electrodes. The transistors have a channel length of 40 μm and width of 11.52 mm ( W / L =288) (detailed fabrication processes are described in the Methods section) with an integrated structured PDMS dielectric (pyramids of 3 μm height, 6 μm base length, 8.85 μm spacing) and a common top gate. Out of two fabricated arrays (total 32 pixels) only one pixel did not show any transistor behaviour from which the yield is roughly estimated to >97%. Transfer curves in the linear ( V SD =−10 V) and saturation regime ( V SD =−100 V) were taken for each of the 15 working pixels on one array at a constant pressure of 11 kPa (capacitance 0.264 nF cm −2 ). It can be seen from the data below that the transistor performance was very uniform in the array. The average mobility measured was 0.09±0.0008, cm 2 V −1 s −1 in the saturation regime and 0.088±0.034 cm 2 V −1 s −1 in the linear regime. The average threshold voltage was −17.1±4.5 V in the saturation regime and −36.7±3.4 V in the linear regime. The larger threshold voltage in the linear regime points to injection limitation at low source-drain voltages, thus requiring a higher charge carrier density to be induced by the gate to lower the injection barrier. The array was able to provide spatially resolved images of light-weight objects of various shapes ( Supplementary Fig. S5 ), such as a paper star weighing only 46 mg ( Fig. 7 ). 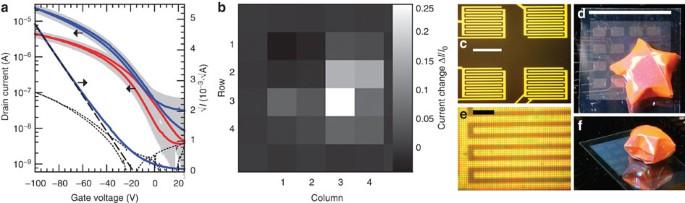Figure 7: Performance and photos of a 4 × 4 pixel array of pressure-sensitive transistors. Channel length is 40 μm, andW/L=288 with a common pyramid-structured (3 μm height, 6 μm base length, 8.85 μm spacing) dielectric and top gate. (a) Transfer curves in the saturation (blue) and linear (red) regime; average data from 15 working pixels taken at a pressure of 11 kPa (capacitance 0.264 nF cm−2). The grey areas indicate the standard deviation. Broken line: fit (taken from −100 to −80 V) to the square of the saturation current for threshold voltage determination. Dotted line: typical (not averaged) gate current. (b) Normalized current change distribution on the sensor array upon placing a light weight (a 46-mg star made from paper) in the lower right corner; seedfor a top view (scale bar, 1 cm), andffor a side view. (c) Microscope picture of 4 pixels right after photoresist lift-off illustrating the source and drain electrodes design (scale bar, 1 mm). (e) Microscope image showing details of 1 pixel of the completed device, taken through the transparent top substrate (scale bar, 200 μm). The small dots are the pyramids in the PDMS dielectric. For an overview with the leads for measurement, seeSupplementary Fig. S6. Figure 7: Performance and photos of a 4 × 4 pixel array of pressure-sensitive transistors. Channel length is 40 μm, and W / L =288 with a common pyramid-structured (3 μm height, 6 μm base length, 8.85 μm spacing) dielectric and top gate. ( a ) Transfer curves in the saturation (blue) and linear (red) regime; average data from 15 working pixels taken at a pressure of 11 kPa (capacitance 0.264 nF cm −2 ). The grey areas indicate the standard deviation. Broken line: fit (taken from −100 to −80 V) to the square of the saturation current for threshold voltage determination. Dotted line: typical (not averaged) gate current. ( b ) Normalized current change distribution on the sensor array upon placing a light weight (a 46-mg star made from paper) in the lower right corner; see d for a top view (scale bar, 1 cm), and f for a side view. ( c ) Microscope picture of 4 pixels right after photoresist lift-off illustrating the source and drain electrodes design (scale bar, 1 mm). ( e ) Microscope image showing details of 1 pixel of the completed device, taken through the transparent top substrate (scale bar, 200 μm). The small dots are the pyramids in the PDMS dielectric. For an overview with the leads for measurement, see Supplementary Fig. S6 . Full size image The sensitivity (8.4 kPa −1 ) of our device in the low-pressure regime <8 kPa in combination with its fast response time (<10 ms) is unprecedented when compared to recent reports on flexible pressure sensors. Sensors based on conductive rubber are mostly limited in response time by their large hysteresis effects [2] , [4] , [25] . Piezoelectric sensors show high dynamic pressure sensitivity but require complex support electronics for sensing true static pressure [40] . Recently, Pang et al. [5] have demonstrated pressure sensors based on interlocked arrays of Pt-coated polymeric nanofibers with high sensitivity but inaccurate response to pressure changes >1 Hz. In this work, we achieved high sensitivity by operating the thin-film transistor in the subthreshold regime. Subthreshold operation has been proposed for lowering the power consumption of integrated circuits, and increasing sensitivity in Si nanowire biosensors and OTFT temperature sensors [41] , [42] . Despite the fact that a large subthreshold regime reduces the switching speed of transistors, surprisingly, our sensor shows no sign of being limited by the transistor speed, as we observed response times in the <10 ms region mainly limited by small residual hysteresis effects of the microstructured PDMS dielectric upon pressure release. During continuous operation at constant source-drain and source-gate voltage, we observed a bias stress effect that causes the source-drain current to decrease during the first 100 s of operation and to stabilize at around 50% of its initial value ( Supplementary Fig. S7 ). However, as can be seen from the stable device operation over >15,000 pressure cycles during 45 min of continuous operation, the bias stress effect does not strongly affect long-term measurements. Moreover, an alternating device operation between on and off states like in the pulse measurements is known to significantly reduce bias stress effects [43] . We have shown that the device also operates well in the bent state, which is required for electronic skin and biomonitoring applications. Although the strong bending response makes our current sensor design interesting as a high-sensitivity flexion sensor in robotics applications [44] , [45] , [46] , it also complicates discrimination between pressure and bending. To reduce the device response to bending, it is necessary to carefully change the device design in order to move the most compressible part, that is, the microstructured PDMS dielectric, into the mechanically neutral plane [4] . The reason is that the bending response has the same underlying mechanism as the pressure response—that is, compression of the structured PDMS. Other effects upon bending, like morphological changes in the polymer semiconductor layer that may lead to an increase in mobility, have been reported previously, but are too small to explain the observed sensitivity [47] . Another possible way to distinguish between bending and pressing would be to use an array of sensors with identical architecture and comparative read-out logic. Our demonstration of high-fidelity human radial artery pulse wave monitoring clearly demonstrates that only a device that combines high pressure sensitivity and fast response time can be used in practical applications like real-time biomonitoring. Being lightweight with low power consumption, our device is suitable for long-term diagnostics. Further development will aim at the further reduction of the power consumption, mainly by reducing the operating voltage. Nevertheless, even with the current device having a thick microstructured PDMS (7 μm), we were able to operate the sensors at below 36 V while maintaining the measurement sensitivity (see Supplementary Fig. S4 ). Therefore, further investigations on reducing the structural dimensions of the PDMS and increasing its dielectric constant by means of incorporating high- k nanoparticles are underway in order to address the high voltage requirement from the fairly low capacitance of the PDMS dielectric. The study on the influence of geometric and bias parameters on pressure sensitivity reveals that it is possible to adjust the device sensitivity both in the low- and in the high-pressure regime, thus enabling tailored pressure sensors for different kinds of applications with different sensitivity requirements. For that matter, the transistor device configuration proves to be advantageous over the capacitor device as it provides two more parameters, that is, source-gate and source-drain voltage, to tune the sensitivity, which can even be changed dynamically. However, there are many more geometric parameters like height and specific shape of the microstructures, which likely also have an influence on the sensitivity. In conclusion, the integration of a microstructured PDMS dielectric and a thin-film polymer semiconductor not only enabled us to fabricate a flexible plastic pressure-sensitive transistor, but we also observed a much improved sensitivity at low pressure as the transistor operates in the subthreshold regime while keeping a very fast response time. Its superior capabilities are demonstrated by the high-fidelity measurements of a human radial artery pulse wave with accuracy and ease of use. Device fabrication Polyimide (Kapton HN 5 mil) substrates were sonicated in deionized water:extran (5 vol%) and rinsed for 10 min with deionized water, followed by rinsing with acetone and isopropanol for 30 s. They were blown dry with a nitrogen gun, and dried for 2 h at 120 °C in a vacuum oven. BCB (Cyclotene 3022-35 from Dow Chemical) was spin-coated at 5,000 r.p.m., soft cured in ambient air on a hotplate set at 120 °C for 1 h and hard cured in a dry nitrogen atmosphere (glovebox) on a hotplate for 25 min at 100 °C, 15 min at 150 °C and 15 h at 220 °C, resulting in a 1 μm thick film with <2 nm root mean square surface roughness determined by atomic force microscopy ( Supplementary Fig. S8 ). The sample was UV ozone treated for 10 min, then soaked for 1 h in a mercaptopropyltrimethoxysilane (MPTMS, Gelest):hexane solution (20 μl:20 ml) for 1 h, rinsed with toluene and methanol, baked at 120 °C for 30 min, briefly sonicated in toluene, rinsed with methanol, and blown dry with a nitrogen gun. Gold drain and source electrodes (40 nm) were thermally evaporated through a shadow mask to give a channel length of 50 μm and a channel width of 16 mm. To remove MPTMS from the channel region, the sample was again UV ozone treated for 10 min, briefly sonicated in toluene, rinsed with ethanol, and blown dry with a nitrogen gun. A polymer semiconductor, PiI2T-Si synthesized as previously described [32] , was spin-coated from a chloroform solution (4 mg ml −1 ) at 1,500 r.p.m. for 60 s and annealed at 160 °C for 1 h in a dry nitrogen atmosphere, resulting in a 70-nm thick film. PDMS (700 nm thickness) was spin-coated from a hexane solution (1:10 wt%) at 5,000 r.p.m. for 120 s and annealed at 120 °C for 1 h. Microstructured PDMS was prepared on ITO-coated PET (Sigma Aldrich 5 mil, 60 Ω sq −1 ) following previously reported procedures [3] . The two parts were laminated together by pressing them against each other and sandwiched between two glass plates and annealing them at 90 °C under 2.5 kPa pressure, then glued at the edges with epoxy adhesive (Devcon 5-minute epoxy) and annealed again inside a nitrogen glovebox for 5 h at 100 °C to remove residual water and oxygen. Wires were attached to the gold source, drain and gate contacts with conductive epoxy (circuit works CW2400). The array fabrication deviates in the steps for substrate preparation and bottom source and drain electrodes as follows. For the sensor array, ~12 μm thick polyimide (HD Microsystems 2525) was spin-coated on a Si carrier wafer followed by BCB planarization and photolithographic patterning of the drain and source electrodes (40 μm in channel length and 11.52 mm in channel width) using dual-layer photoresists (Shipley 3612 and LOL2000). Gold was then thermally evaporated followed by a N -methyl-2-pyrrolidone bath for lift-off. After surface treatment, the polymer semiconductor was subsequently deposited followed by the PDMS protection layer and the lamination of microstructured PMDS (pyramids with 3 μm height, 6 μm base length, and 8.85 μm spacing) supported on ITO-coated PET as the gate electrode. Device characterization Transistor measurements were carried out with a Keithley 4200-SCS. Pressure was applied and measured either with a high-precision motorized z-stage (Newmark Systems NVS-12) in combination with force gauge (Mark-10 BG05) or by placing different weights onto the device. The area was defined by a small glass piece (0.36 cm 2 ). The interface trap density was estimated from the subthreshold slope S =32 V per decade (derived from the transfer characteristics between −20 and −55 V) and the dielectric capacitance C diel =0.273 nF cm −2 measured at 46 kPa. The subthreshold slope is given by , with the interface trap capacitance C it , which is related to the interface trap density D it = C it / e (ref. 48 ). Measurements on the bent device were done while the device was attached to various round objects with different curvatures. Cycling and response time measurements were done with the motorized z-stage while the device was operated at constant source-drain and source-gate voltage, each in the range from −36 to −100 V. The sensor signal was recorded with a personal computer-based oscilloscope (Velleman Instruments PCSGU250) as the voltage drop over a 9-MΩ resistance connected in series between the OTFT source and ground. Since the force gauge response time was too slow to accurately follow and record the pressure changes in the cycling and response time measurements, the applied pressure was calculated from the z-stage movement parameters initial and final velocity, acceleration and deceleration. Radial artery pulse wave measurements were carried out by attaching the pressure sensor to the wrist just above the spot where the pulse was detectable with the structured PDMS side facing the skin. Applied voltage and signal recording was the same as for the cycling and response time measurements. For the averaged signal used for determination of the arterial stiffness diagnostic parameters, the internal averaging function of the oscilloscope was used. Capacitance calculation The capacitance of one pyramid between two parallel electrodes was calculated by the following formula: with , where b is the base length, h the height of the pyramid, ε 0 the vacuum permittivity, ε 1 the dielectric constant of PDMS and ε 2 the dielectric constant of air. ε 1 was experimentally measured as 2.34 by spin-coating the same PDMS formulation as used for the structures on a Si wafer, evaporating Au electrodes on top and measuring the capacitance and the thickness of the film. ε 2 is assumed to be 1. By knowing the capacitance of one pyramid, it is then straightforward to calculate the average capacitance per area for the different structure spacings. The dimensions (height, base-length, and spacing) of the fabricated pyramid structures were determined from SEM pictures and averaged over at least six individual features. The base-film thickness was determined by profilometer measurements (DekTak). How to cite this article: Schwartz, G. et al. Flexible polymer transistors with high pressure sensitivity for application in electronic skin and health monitoring. Nat. Commun . 4:1859 doi:10.1038/ncomms2832 (2013).